Gate control of the electron spin-diffusion length in semiconductor quantum wells The spin diffusion length is a key parameter to describe the transport properties of spin polarized electrons in solids. Electrical spin injection in semiconductor structures, a major issue in spintronics, critically depends on this spin diffusion length. Gate control of the spin diffusion length could be of great importance for the operation of devices based on the electric field manipulation and transport of electron spin. Here we demonstrate that the spin diffusion length in a GaAs quantum well can be electrically controlled. Through the measurement of the spin diffusion coefficient by spin grating spectroscopy and of the spin relaxation time by time-resolved optical orientation experiments, we show that the diffusion length can be increased by more than 200% with an applied gate voltage of 5 V. These experiments allow at the same time the direct simultaneous measurements of both the Rashba and Dresselhaus spin-orbit splittings. The length scale over which the travelling electron spin keeps the memory of its initial orientation is known as the spin-diffusion length [1] , [2] , [3] , [4] , [5] , which is a critical parameter for many spintronic devices [6] , [7] , [8] , [9] , [10] , [11] , [12] . In semiconductors, this distance is closely linked to spin relaxation and spin transport properties of conduction electrons, which in turn depend on the spin-orbit interaction. In quantum wells made of III–V semiconductors such as the model GaAs/AlGaAs system, the conduction-band (CB) spin splitting has two origins: the first one, called Bulk Inversion Asymmetry (BIA) or Dresselhaus term, is the consequence of the combined effect of spin-orbit interaction and the lack of crystal inversion symmetry [13] , [14] . The second contribution to the spin splitting, called Structural Inversion Asymmetry (SIA) or Rashba term, exists if the quantum well experiences an electric field [15] , [16] . The interplay of these two terms can yield longer relaxation times for electron spins oriented along some specific crystallographic directions [17] , [18] or original effects, such as Spin helix [19] , [20] . After a few years of debates, it was recently shown that the Rashba-induced conduction-band spin splitting requires the application of a real electric field in the structure (through asymmetric doping or PIN structures), whereas CB potential gradients, which also break the inversion symmetry, yield negligible small Rashba splitting [13] , [21] , [22] . Thanks to the unique relative orientation of the Dresselhaus and Rashba fields in (111)-oriented semiconductor quantum wells, we show here that the electron spin-diffusion length can be electrically controlled, a feature that was never demonstrated before. Moreover, the all-optical measurement of the electric field dependence of the electron spin-relaxation time and the spin-diffusion coefficient allows us to get a direct determination of both the Dresselhaus and Rashba coefficients independently. Electric field effect on the spin-diffusion coefficient Spin-polarized electrons are photogenerated by exciting the non-intentionally doped quantum wells using a circularly polarized laser. The quantum wells are embedded into an NIP structure in which a reverse bias V can be applied, yielding the variation of the electric field E experienced by the spin-polarized electrons ( Fig. 1 ). The spin-diffusion length L s is simply linked to the spin lifetime T s and the spin-diffusion coefficient D s through (refs 23 , 24 ). We performed an optical measurement of the spin-diffusion constant D s by using the Transient Spin-Grating technique [23] , and we measured the electron spin lifetime T s by the time-resolved photoluminescence spectroscopy [25] (see Methods). 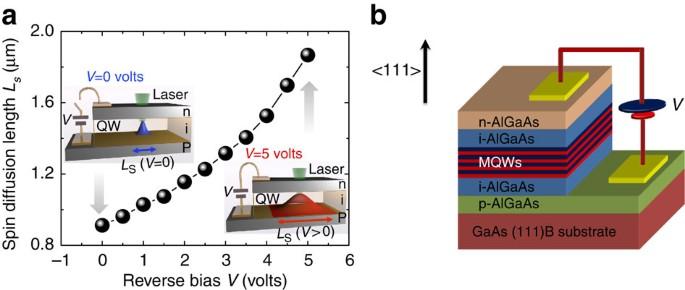Figure 1:Gate control of the spin-diffusion length. (a) Variation of the spin-diffusion lengthas a function of the reverse biasVapplied on the NIP device obtained from combined measurements of the electron-spin lifetimeTsand the electron spin-diffusion constantDs. Insets: schematics of the gate control of the electron spin-diffusion lengthLsin a (111)-oriented GaAs/AlGaAs quantum well. The red (V=5 volts) and blue (V=0) surfaces illustrate the spatial distribution of the spin density in the quantum well plane under laser excitation. (b) Schematic representation of the NIP junction with 20 GaAs/Al0.3Ga0.7As QWs embedded in its intrinsic region. The growth axiszcorresponds to the <111> direction. Figure 1: Gate control of the spin-diffusion length . ( a ) Variation of the spin-diffusion length as a function of the reverse bias V applied on the NIP device obtained from combined measurements of the electron-spin lifetime T s and the electron spin-diffusion constant D s . Insets: schematics of the gate control of the electron spin-diffusion length L s in a (111)-oriented GaAs/AlGaAs quantum well. The red ( V =5 volts) and blue ( V =0) surfaces illustrate the spatial distribution of the spin density in the quantum well plane under laser excitation. ( b ) Schematic representation of the NIP junction with 20 GaAs/Al 0.3 Ga 0.7 As QWs embedded in its intrinsic region. The growth axis z corresponds to the <111> direction. Full size image A spin-density wave with wavelength Λ is created by the interferences of two cross-polarized pump laser beams ( Fig. 2 ). The modulus of wave vector q of the spin grating is equal to q =2 π / Λ . Figure 3a displays the decay of the spin-grating signal as a function of the delay between the pump and the probe laser pulses for a reverse bias V =1 volt. 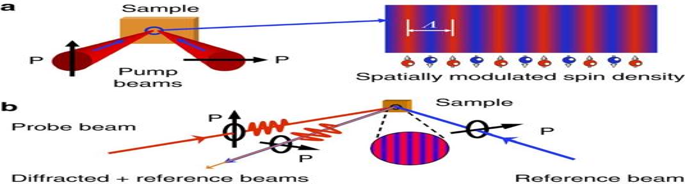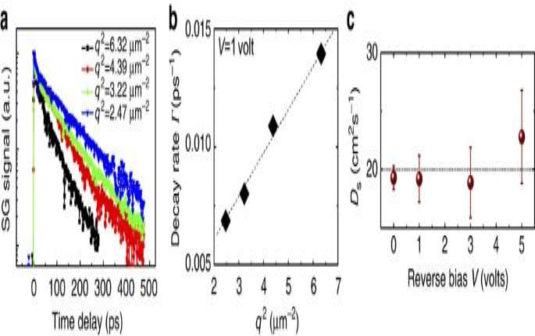Figure 3: Electron spin diffusion. (a) Time evolution of the spin-grating (SG) signal as a function of the delay between the pump and the probe laser pulses forV=1 volt. To separate the effects of spin diffusion and spin relaxation, the grating decay rateis measured for different grating wave vectorsqby changing the phase mask period (see Methods). (b) Decay rateΓof the SG signal for a reverse biasV=1 volt. (c) Spin-diffusion coefficientDsas a function of the gate voltageV.The error bars correspond to the uncertainties of the slope determination (seeFig. 3b). Figure 2: Transient spin grating. (a) Schematic of the transient spin-grating technique based on the interferences of the two cross-polarized pump beams yielding a spatially modulated spin density in the quantum well plane with a periodΛ. (b) The spin-grating signal detected with a heterodyne technique based on a reference beam is recorded as a function of the time delay between the pump and the probe pulses (see Methods). The decay rate Γ of this spin-density wave is simply given by [23] , [26] : Figure 2: Transient spin grating. ( a ) Schematic of the transient spin-grating technique based on the interferences of the two cross-polarized pump beams yielding a spatially modulated spin density in the quantum well plane with a period Λ . ( b ) The spin-grating signal detected with a heterodyne technique based on a reference beam is recorded as a function of the time delay between the pump and the probe pulses (see Methods). Full size image Figure 3: Electron spin diffusion. ( a ) Time evolution of the spin-grating (SG) signal as a function of the delay between the pump and the probe laser pulses for V =1 volt. To separate the effects of spin diffusion and spin relaxation, the grating decay rate is measured for different grating wave vectors q by changing the phase mask period (see Methods). ( b ) Decay rate Γ of the SG signal for a reverse bias V =1 volt. ( c ) Spin-diffusion coefficient D s as a function of the gate voltage V. The error bars correspond to the uncertainties of the slope determination (see Fig. 3b ). Full size image To separate the effects of spin diffusion and spin relaxation, the grating decay rate Γ is measured for different grating wave vectors q by changing the phase mask period (see Methods). Performing the measurement of Γ for different grating periods (and hence q 2 values) yields an accurate determination of D s , whose dependence on the gate voltage has never been investigated. Figure 3b displays the variation of Γ as a function of q 2 for an applied reverse bias V =1 volt. We measured a spin-diffusion coefficient D s ~20 cm 2 s −1 . We performed the same experiments for different applied gate voltages. Figure 3c shows that the spin-diffusion coefficient D s is almost constant whatever the applied vertical electric field is; this value is consistent with previously reported spin-diffusion coefficients in non-intentionally doped GaAs quantum wells [27] , [28] , [29] . Gate voltage variation of the spin lifetime In order to obtain the electric field dependence of the spin-diffusion length L s , we need to determine the variation of the spin lifetime T s measured independently as a function of the gate voltage. The striking feature of (111)-oriented quantum well is that the electron spin-relaxation time can be electrically controlled for any electron-spin orientation [25] , [30] . The accurate determination of the electric field dependence of the electron spin lifetime T s has been obtained from spin-polarized time-resolved photoluminescence spectroscopy ( Fig. 4a,b ). 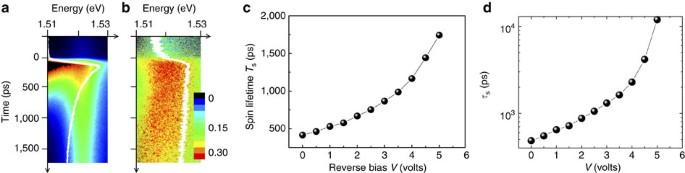Figure 4: Spin Lifetime in the gate-control device. (a) Photoluminescence intensity (colour code in arbitrary units) as a function of both time and photon energy for a reverse biasV=5 volts. The white curve represents the PL intensity as a function of time when the emission is spectrally integrated. The decay time of this PL dynamics corresponds to the electron lifetimeτ. (b) PL circular polarization degreePc(colour code fromPc=0 toPc=0.30) as a function of both time and photon energy for a reverse biasV=5 volts.Pc=(I+−I−)/(I++I−), whereI+andI−are the PL circular components, respectively, co- and counter-polarized with the incident laser beam. The white curve representsPcas a function of time when the emission is spectrally integrated. The decay time of thisPcdynamics corresponds to the electron spin-relaxation timeτs. (c) Gate control of the electron spin lifetimeTs. (d) Gate control of the spin-relaxation timeτs. Figure 4c displays the dependence of T s as a function of the applied voltage, where 1 /T s =1 /τ s +1 /τ ; both the electron spin-relaxation time τ s and the electron lifetime τ have been measured for each value of the reverse bias V . The electron-spin lifetime can be controlled with the applied electric field with an increase by a factor of about four when the reverse bias varies from 0–5 volts. We checked that the same gate voltage dependence of T s was measured by time-resolved Kerr rotation experiments performed on the same set-up as the spin-grating measurements. Figure 4: Spin Lifetime in the gate-control device. ( a ) Photoluminescence intensity (colour code in arbitrary units) as a function of both time and photon energy for a reverse bias V =5 volts. The white curve represents the PL intensity as a function of time when the emission is spectrally integrated. The decay time of this PL dynamics corresponds to the electron lifetime τ . ( b ) PL circular polarization degree P c (colour code from P c =0 to P c =0.30) as a function of both time and photon energy for a reverse bias V =5 volts. P c =( I + − I − )/( I + + I − ), where I + and I − are the PL circular components, respectively, co- and counter-polarized with the incident laser beam. The white curve represents P c as a function of time when the emission is spectrally integrated. The decay time of this P c dynamics corresponds to the electron spin-relaxation time τ s . ( c ) Gate control of the electron spin lifetime T s . ( d ) Gate control of the spin-relaxation time τ s . Full size image Figure 1a presents the resulting variation of the spin-diffusion length as a function of the applied voltage. It increases by more than a factor two when the amplitude of the electric field increases, reaching a value L s ~1.8 μm for | E |~55 kV cm −1 corresponding to V =5 volts. These results provide the proof of concept that the spin diffusion length can be electrically controlled in semiconductors. Here the increase of L s is limited by the electron lifetime τ because for V >4 volts the spin relaxation time is much longer than τ in these non-intentionally doped quantum wells ( Fig. 4d ). In n-doped (111) quantum wells, which are of interest for spintronic applications [11] , [12] , we expect a much larger variation of L s with the applied voltage that will be no more limited by the electron lifetime. In that case, the variation of L S with the voltage V will just depend on the square root of the electron spin-relaxation time τ s , which can vary by several orders of magnitude with V [25] , [30] . The all-optical measurements of both the spin relaxation dynamics and the electron spin diffusion allow us to get a precise and independent determination of the Dresselhaus and Rashba coefficients, which are the key parameters to control and manipulate the carrier spins in semiconductors. Despite the numerous experimental and theoretical investigations, the reported values of the Dresselhaus and Rashba coefficients in GaAs vary strongly, ranging from | γ |=3 to 35 eV Å 3 for Dresselhaus [29] , [31] , [32] , [33] , [34] , [35] and r 41 from 5–10 e Å 2 for Rashba [13] , [29] , [36] . Most of the techniques used so far give only the ratio between the Rashba and Dresselhaus terms or allow the determination of only one type of spin splitting. They also require the investigation of n-doped quantum wells with electrical contacts [31] , [37] , [38] . The technique presented here, which yields the determination of both Dresselhaus and Rashba spin-orbit (SO) splitting in the same sample, could be applied for any doped or undoped III–V or II–VI cubic semiconductor quantum wells. The only requirement is to grow the structures on (111)-oriented substrates. In a (111) quantum well, where the momentum component along the growth axis z is quantized, the spin precession vector Ω(k) due to the Dresselhaus (BIA) term for the lowest electron subband is written as [39] : where is the averaged squared wave vector along the growth direction, k // is the in-plane wave vector ( ) and γ is the Dresselhaus coefficient [40] . The weaker cubic terms in the Hamiltonian have been neglected here (at 50 K for a well width L W =15 nm, the average cubic Dresselhaus term is 10 times weaker than the linear one). For an electric field applied along the growth axis, the SIA (Rashba) component writes: where α =2 r 41 E is the Rashba coefficient ( E is the electric field amplitude and r 41 is a positive constant [13] ). In contrast to (001) or (110)-oriented quantum wells, equations (2) and (3) show that the BIA and SIA vectors have exactly the same direction in the (111) QW plane and the same electron momentum dependence [25] . Thus the total spin precession vector has the form: This spin precession vector will drive the well-known dominant D’yakonov–Perel electron spin-relaxation mechanism in the quantum well. The corresponding spin-relaxation time is given by [14] , [41] : where is the mean square precession vector in the plane perpendicular to the electron spin direction (which is here along z ) and is the electron momentum-relaxation time [41] . Substitution of equation (4) into equation (5) and taking the thermal average yields: This means that the measurement of both the electron spin-relaxation time τ s and the electron momentum-relaxation time as a function of the applied electric field gives a direct determination of both the Dresselhaus and Rashba coefficients. The electron momentum-relaxation time can be obtained from the spin-grating experimental results presented above. On the basis of the Einstein relation, we have , where D e is the charge diffusion constant, μ the electron mobility and m* the electron effective mass. For undoped quantum wells, the electron spin-diffusion coefficient is equal to the electron diffusion coefficient ( D e =D s ) [29] . As a consequence, the spin-diffusion coefficient D s measured in Figure 3c allows us to measure ; we find ~200 fs with no variation with the applied electric field within the experimental uncertainties. Using this value and the measured variation of the electron spin-relaxation time τ s as functions of the applied electric field, we have plotted in Fig. 5 the curve β +2 r 41 E using equation (6). From the slope and the intercept of this curve, we get straightforwardly the Rashba and Dresselhaus coefficients ( =2.5 × 10 16 m −2 is obtained in the framework of a finite QW barrier calculation [31] ). We find β =1.06±0.1 × 10 −3 eV nm yielding a Dresselhaus coefficient γ =18±2 eV Å 3 , whereas the calculated value for GaAs is γ ≅ 24 eV Å 3 (refs 13 , 35 ). From the slope of the curve in Fig. 5 , we get the Rashba coefficient r 41 =7±1 e Å 2 , consistent with the calculated value r 41 =5.2 e Å 2 (ref. 13 ). 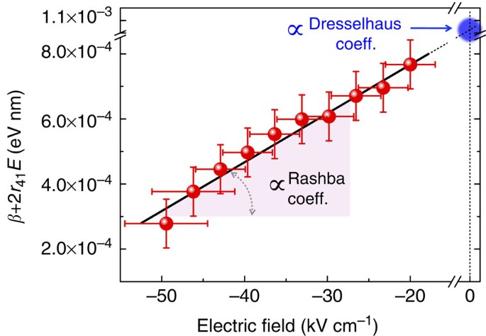Figure 5: Simultaneous measurement of the Dresselhaus and Rashba coefficients. Variation ofβ+2r41Eas a function of the applied electric fieldEin the device. The red triangle schematically represents the slope of this function used to extract the Rashba coefficientr41. The intercept ofβ+2r41Ewith the ordinate axis givesβ(β=4γ‹Kz2›/), whereγis the Dresselhaus coefficient. Thexaxis error bars have been calculated from the uncertainties on the measured stark shift. Theyaxis error bars correspond to the uncertainties on the measurement of the spin-relaxation timeτsand momentum-relaxation time. Figure 5: Simultaneous measurement of the Dresselhaus and Rashba coefficients. Variation of β +2 r 41 E as a function of the applied electric field E in the device. The red triangle schematically represents the slope of this function used to extract the Rashba coefficient r 41 . The intercept of β +2 r 41 E with the ordinate axis gives β ( β= 4 γ ‹ K z 2 ›/ ), where γ is the Dresselhaus coefficient. The x axis error bars have been calculated from the uncertainties on the measured stark shift. The y axis error bars correspond to the uncertainties on the measurement of the spin-relaxation time τ s and momentum-relaxation time . Full size image In conclusion, we have demonstrated for the first time the gate control of the electron spin-diffusion length in a semiconductor nanostructure. In addition to its interest for spintronic devices, this effect allows an accurate determination of both Dresselhaus and Rashba coefficients. It can be applied in any zinc-blende III–V and II–VI quantum wells and in wurtzite (0001) nanostructures as well [42] , as the principle relies only on symmetry considerations. We emphasize that this electrical control of the spin-diffusion length is effective whatever the injected carrier spin orientation is. This opens an avenue for spin manipulation and control in semiconductors. Sample The investigated sample is grown on (111)B-oriented semi-insulating GaAs substrate using molecular beam epitaxy. The (111)B substrate is misoriented 3° towards <111>A. The layer sequence of the NIP structure is: substrate/200 nm GaAs buffer/500 nm p-doped ( p =1.2 × 10 18 cm −3 ) GaAs/100 nm Al 0.3 Ga 0.7 As barrier/MQW/70 nm Al 0.3 Ga 0.7 As barrier/10 nm n-doped ( n =2.8 × 10 18 cm −3 ) GaAs ( Fig. 1b ). The Multiple Quantum Well (MQW) consists of 20 periods of GaAs/Al 0.3 Ga 0.7 As quantum wells with well width and barrier width L W =15 nm and L B =12 nm, respectively. The reverse bias voltage ( V ) is applied between the unetched top n-contact and the chemically etched p-contact. Spin relaxation and spin transport measurements In the Transient Spin-Grating experiment, the laser pulses are generated by a mode-locked Ti:sapphire laser with 120 fs pulse width and 76 MHz repetition frequency and are split into primary pump and probe beams with an average power of 5 and 0.5 mW, respectively ( Fig. 2a ). The wavelength is set to get the maximum signal of Kerr rotation for each reverse bias V through the standard time-resolved Kerr rotation technique [18] . Both pump and probe beams are focused on a phase mask ( StockerYale. Inc. ) with a period d . The phase mask splits each of the primary beams by diffraction into the m =±1 orders. The interference between the two pump beams with orthogonal linear polarization yields a spatially modulated circular polarization across the excitation spot. According to the optical interband selection rules, this interference pattern will generate a periodical spin density, called the spin grating. The period Λ of the transient spin grating is simply , where f 1 and f 2 are the focal lengths of two spherical mirrors. In our set-up, the focal lengths of the first and second spherical mirrors are fixed at f 1 = f 2 =30.4 cm. The spot sizes of both pump and probe beams are ~200 μm. The wave vector modulus q of the spin grating is equal to with a phase mask of d =5 μm. Phase masks with d =5, 6, 7 and 8 μm are used. A delayed probe beam with vertical linear polarization is incident on the spin grating and the corresponding diffracted beam is detected as a function of the time delay between the pump and the probe pulses ( Fig. 2b ). A heterodyne detection of the transient grating is implemented using a reference beam with horizontal linear polarization incident on the sample [43] . The four beams (two pump beams, probe and reference beams) are arranged in the boxcar geometry [43] . In this scheme based on two lock-in amplifiers, the pump beam is modulated by a photoelastic modulator with a frequency of 100 kHz, and the probe beam is mechanically chopped at 60 Hz. This heterodyne configuration yields an increase in the signal to noise ratio by more than two orders of magnitude. The spin-grating signal (proportional to the modulus the electric field of the diffracted probe beam) is simply given by I SG =A exp(− Γ Δ t ), where A is a constant, Γ is the decay rate of the spin grating and Δt is the time delay between the pump and probe pulses. The electron spin-relaxation time τ s and electron lifetime τ are measured from time and polarization resolved photoluminescence experiments using circularly polarized picosecond Ti:Sapphire laser pulses and a synchroscan Streak camera with an overall time resolution of 8 ps [44] . All the measurements are performed at T =50 K. How to cite this article: Wang, G. et al . Gate control of the electron spin-diffusion length in semiconductor quantum wells. Nat. Commun. 4:2372 doi: 10.1038/ncomms3372 (2013).